Long non-coding RNAs and enhancer RNAs regulate the lipopolysaccharide-induced inflammatory response in human monocytes Early reports indicate that long non-coding RNAs (lncRNAs) are novel regulators of biological responses. However, their role in the human innate immune response, which provides the initial defence against infection, is largely unexplored. To address this issue, here we characterize the long non-coding RNA transcriptome in primary human monocytes using RNA sequencing. We identify 76 enhancer RNAs (eRNAs), 40 canonical lncRNAs, 65 antisense lncRNAs and 35 regions of bidirectional transcription (RBT) that are differentially expressed in response to bacterial lipopolysaccharide (LPS). Crucially, we demonstrate that knockdown of nuclear-localized, NF-κB-regulated, eRNAs ( IL1β-eRNA ) and RBT ( IL1β-RBT46 ) surrounding the IL1β locus, attenuates LPS-induced messenger RNA transcription and release of the proinflammatory mediators, IL1β and CXCL8. We predict that lncRNAs can be important regulators of the human innate immune response. Genome-scale transcriptional responses of protein-coding genes following lipopolysaccharide (LPS)-induced activation of the innate immune response in human monocytes and monocytic cell lines have been extensively studied using both microarrays [1] and serial analysis of gene expression [2] , [3] . These studies have clearly demonstrated the induction of many members of proinflammatory cytokines (for example, IL1β, CXCL8, IL6 and tumor necrosis factor alpha ( TNFα )), chemokines and cell surface markers in response to Toll-like receptor 4 (TLR4) signalling [3] . Significantly, the advent of next-generation sequencing technology has allowed for an unbiased investigation of the full repertoire of transcription from both coding and non-coding regions of the genome. Evidence for pervasive transcription across the genome now exists in the form of large sequenced cDNA libraries [4] , histone modification chromatin immunoprecipitation (ChIP)-seq data sets [5] , [6] and messenger RNA (mRNA) sequencing (RNA-seq) data sets [7] , [8] as part of multi-centre collaborative projects such as FANTOM, ENCODE and the HumanBodyMap. These data sets have revealed the presence of a large number of non-coding RNAs, which display both tissue- and developmental time point-specific transcription [6] , [7] , [9] . Several classes of non-coding RNAs have been characterized, and some, such as microRNAs (miRNA), have been well studied. Indeed, miRNAs have been shown to play a role in the cellular response to LPS [10] , [11] . However, the regulatory potential of long non-coding RNAs (lncRNAs) has emerged only recently (reviewed in ref. 12 ). While the function of the majority of these RNA species is yet to be elucidated, there is increasing evidence to support their diverse mechanistic roles. Some act as structural molecules in the recruitment of histone-modifying enzymes either in cis or trans (reviewed in ref. 12 ), while others are transcribed from enhancer regions (eRNAs [13] ), facilitating transcription of protein-coding genes via RNA-dependent or RNA-independent mechanisms [14] . Studies in mouse macrophages and bone marrow-derived dendritic cells have revealed the regulation of intergenic transcription in response to proinflammatory signals (LPS and IFNγ) [6] , [15] , [16] . Interestingly, transcription from intergenic loci is not always coincident with canonical promoter histone modification signatures. Indeed, a large proportion is derived from regions of the genome that contain a high H3K4me1/H3K4me3 ratio, suggesting that lncRNAs are commonly derived from enhancer elements (eRNAs) [15] , [17] . Transcriptional complexity is further increased when we consider the presence of non-polyadenylated, bidirectional transcripts produced from additional sets of enhancers [18] . While the function of lncRNAs in the human innate immune response is not well described, recent studies have begun to elucidate the mechanism of action of some mouse lncRNAs. Thus, Rapicavoli et al . [19] identified a pseudogene for ribosomal protein S15a (Rsp15a), renamed Lethe, that negatively regulates the inflammatory response through an interaction with RelA (p65), a component of the NF-κB complex [19] . Similarly, Carpenter et al . [20] showed rapid induction in the expression of a lincRNA localized ~50 Kb downstream of COX2 (named lincRNA-Cox2) that mediates both the activation and repression of inflammatory response through interaction with the nuclear ribonucleoprotein A/B and A2/B1. A single publication in human macrophages derived from human monocytic THP-1 cells has identified a lincRNA named TNFα and heterogeneous nuclear ribonucleoprotein L-related immunoregulatory LincRNA from a microarray screen that regulated the inflammatory response [21] . While these studies have been valuable in determining lncRNA regulation in response to LPS in cells of the mouse innate immune system, sequencing studies have not yet been performed in humans. In contrast to the observed global human–mouse transcriptional conservation of protein-coding genes [22] , rapid transcriptional turnover of a vast number of lncRNAs in rodent species suggests the evolution of lineage-specific transcription [23] . This provides the impetus to use human cells to relate lncRNA transcription to human immune function. In this study, we aim to characterize the unexplored aspects of non-coding transcription in cells of the human innate immune system. Specifically, using ab initio transcript assembly of a deeply sequenced RNA data set, we examine the response of lncRNAs to TLR4 signalling through LPS stimulation. By integration of publically available H3K4me1 and H3K4me3 ChIP-seq data from the ENCODE project, we estimate the proportion of LPS-regulated lncRNAs that are derived from enhancer elements (eRNAs) and determine how changes in expression correlate with changes in proximal protein-coding mRNA expression. We also characterize the expression of bidirectional transcripts, a class of elements that have not yet been examined in the innate immune response and use knockdown experiments to determine the functional role of lncRNAs. Our data demonstrate that many lncRNAs in human monocytes show differential expression in response to LPS stimulation—a subset of which are derived from uni- and bidirectional enhancer regions that coexpress with neighbouring inflammatory mediators. Interestingly, knockdown of an eRNA ( IL1β-eRNA ) and a region of bidirectional transcription ( IL1β-RBT46 ) selectively attenuates LPS-induced expression and release of the proinflammatory mediators, IL1β and CXCL8. This suggests a general role for lncRNAs in the regulation of the innate immune response and the release of inflammatory mediators in human monocytes. RNA sequencing shows LPS induction of innate immunity LPS stimulation produced significant increases in the release of the inflammatory mediators CXCL8 and TNFα ( Fig. 1b ), confirming activation of the immune response. Analysis of RNA-seq data for Ensembl (version 66)-annotated mRNAs confirmed this activation at the transcriptional level. A total of 1,621 protein-coding genes were differentially expressed on LPS stimulation at a false discovery rate (FDR)<0.05 and fold change>2 ( Supplementary Fig. 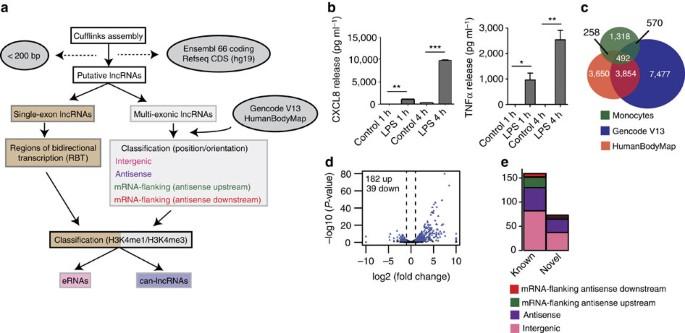Figure 1: LncRNA expression is regulated by LPS in human monocytes. (a) Pipeline for predicting lncRNAs from cufflinks assembled transfrags. HumanBodyMap=lincRNAs predicted in ref.2. Can-lncRNAs=canonical lncRNAs characterized by a low H3K4me1/H3K4me3 ratio. eRNAs characterized by a high H3K4me1/H3K4me3 ratio. (b) Release of CXCL8 and TNFα measured by ELISA shows activation of the innate immune response. Data are the mean±s.e.m. of four independent experiments. Statistical significance was determined using a Studentt-test where *P<0.05, **P<0.01 and ***P<0.001. (c) Overlap of lncRNAs in monocytes, Gencode v13 and lncRNAs from the HumanBodyMap catalogues. (d) Volcano plot displaying differentially expressed lncRNAs (n=4 in each group). Differential expression analysis was performed using a test based on the negative binomial distribution implemented in DESeq. LncRNAs that are significant at an FDR<0.05 are displayed in blue. (e) Breakdown of differentially expressed lncRNAs based on positional classifications. 1a and Supplementary Table 1 ; 1,045 upregulated, 576 downregulated). Further cross-platform analysis revealed that fold changes determined by RNA-seq correlated well with those from microarray-based analysis of the same data set (see Supplementary Fig. 1b online; r =0.74) and both methods called similar sets of genes as differentially expressed (hypergeometric test; P =1.32 × 10 −11 ). A total of 534 genes were called by both methods (415 upregulated, 115 downregulated, 4 incongruent), with 530 representing a robust set of inflammation-regulated genes. As expected, the upregulated genes from this set were significantly enriched (FDR<0.05) in KEGG pathways involved in the inflammatory response including ‘Toll-like receptor signalling’, ‘cytokine–cytokine receptor signalling’ and ‘chemokine signalling pathway’ (see Supplementary Fig. 1c online). There were no significantly enriched pathways in downregulated genes. This initial evaluation of the data revealed that we could accurately recapitulate the known transcriptional response of monocytes to LPS stimulation using our RNA-seq data set. Figure 1: LncRNA expression is regulated by LPS in human monocytes. ( a ) Pipeline for predicting lncRNAs from cufflinks assembled transfrags. HumanBodyMap=lincRNAs predicted in ref. 2 . Can-lncRNAs=canonical lncRNAs characterized by a low H3K4me1/H3K4me3 ratio. eRNAs characterized by a high H3K4me1/H3K4me3 ratio. ( b ) Release of CXCL8 and TNFα measured by ELISA shows activation of the innate immune response. Data are the mean±s.e.m. of four independent experiments. Statistical significance was determined using a Student t -test where * P <0.05, ** P <0.01 and *** P <0.001. ( c ) Overlap of lncRNAs in monocytes, Gencode v13 and lncRNAs from the HumanBodyMap catalogues. ( d ) Volcano plot displaying differentially expressed lncRNAs ( n =4 in each group). Differential expression analysis was performed using a test based on the negative binomial distribution implemented in DESeq. LncRNAs that are significant at an FDR<0.05 are displayed in blue. ( e ) Breakdown of differentially expressed lncRNAs based on positional classifications. Full size image RNA sequencing reveals expression of novel lncRNAs Computational analysis of a set of predicted transcript models as described in Fig. 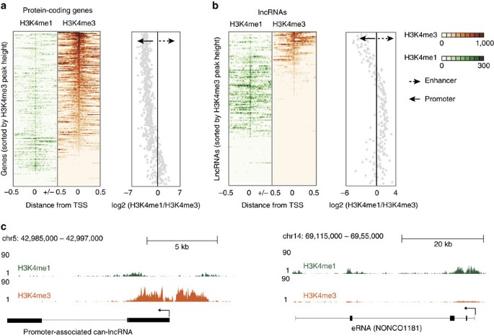Figure 2: LncRNAs can be distinguished by canonical promoter and enhancer chromatin signatures. (a) H3k4me3 and H3K4me1 binding across a 1 Kb interval centred on the transcription start site of expressed protein-coding genes. Profiles are sorted based on the height of the H3K4me3 peak. Also provided is a plot of the H3K4me1/H3K4me3 log2(ratio) at each TSS (mean over interval). (b) H3k4me3 and H3K4me1 binding across a 1 Kb interval centred on the transcription start site of differentially expressed lncRNAs. Profiles are sorted on the height of the H3K4me3 peak. Also provided is a plot of the H3K4me1/H3K4me3 log2(ratio) at each TSS (mean). (c) Example of a lncRNA with a canonical promoter-like chromatin signature (can-lncRNA, left) and a lncRNA with an enhancer signature (eRNA, right). Figures were produced using the UCSC genome browser. 1a identified 2,607 multi-exonic monocyte-derived lncRNA genes (see Supplementary Table 2 online). An additional 69 regions of bidirectional transcription (RBT) were also discovered (see later). As lncRNA transcript models are often fragmentary, we did not consider multiple transcripts of the same gene and the term lncRNA therefore refers to a single consensus gene model. Of these assembled genes, 1,318 (50%) novel lncRNAs had not been previously identified in Gencode v13 or HumanBodyMap lncRNA sets, potentially reflecting monocyte and/or LPS specificity ( Fig. 1c ). We found that lncRNAs were significantly shorter (KS test; D =0.41, P <1 × 10 −16 ), had fewer exons (Wilcoxon rank sum test; W =8.2 × 10 6 , P <1 × 10 −16 ) and were more lowly expressed than protein-coding genes (KS test; D =0.41, P <1 × 10 −16 ) (see Supplementary Fig. 2a–c online), in line with previous findings [7] , [8] . The mean fragments per kilobase exon per million reads mapped (FPKM), length (Kb) and exon number for lncRNAs (versus mRNAs) was 2.14 (7.03), 2.48 (7.93) and 3 (11), respectively. Furthermore, monocytic lncRNAs (based on the 1,318 novel lncRNAs) did not show evidence for coding capacity (see Supplementary Fig. 2d online). Nevertheless, due to low expression levels and potential for fragmentary gene models, we cannot exclude the possibility that we include genes that encode small peptides in our downstream analyses. As described in Fig. 1a , we operationally classified lncRNAs based on their proximity and relative orientation to protein-coding annotations (Ensembl 66). The classifications we used were as follows: antisense (overlapping a protein-coding gene locus on the opposite strand), intergenic (>5 Kb from a protein-coding gene) and mRNA-flanking (<5 Kb from a protein-coding gene (upstream/downstream and sense/antisense)). The distribution of lncRNAs among the different classes was: intergenic (55%), antisense (26%), mRNA flanking (19%=antisense upstream (8%)+sense upstream (4%)+antisense downstream (2%)+sense downstream (5%) (see Supplementary Table 2 ). Those lncRNAs classified as sense upstream or sense downstream were removed from further analyses due to our inability to accurately resolve true ‘sense’ lncRNAs from expression emanating from neighbouring protein-coding loci. LPS induced widespread changes in lncRNA expression We hypothesized that along with many mRNAs and miRNAs, lncRNAs respond to activation of the immune response. 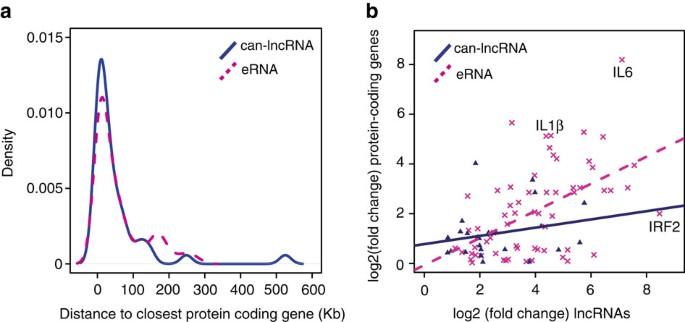Figure 3: eRNA expression correlates with protein-coding gene expression. (a) Distribution of distances from the closest expressed protein-coding gene for eRNAs and can-lncRNAs. (b) Correlation between absolute fold changes for eRNAs and can-lncRNAs with their nearest expressed protein-coding gene neighbour. Following LPS stimulation, we found that 221 out of 989 robustly expressed (FPKM>1) lncRNAs were differentially expressed (see Supplementary Table 3 ). We observed 182 up and 39 downregulated lncRNAs ( Fig. 1d ), of which 76 were from the novel lncRNAs identified in primary human monocytes. The majority of differentially expressed lncRNAs were located >5 Kb from protein-coding annotations with class representation in the order of their proportion being the following: intergenic (51%), antisense (33%) and mRNA-flanking lncRNA (antisense upstream (11%) and antisense downstream (5%)) ( Fig. 1e ). qRT–PCR analysis of a subset of differentially expressed lncRNAs confirmed our RNA-seq results with 14/18 (78%) validated using this method ( Supplementary Fig. 3 ). Of note, only 2 of the 221 differentially expressed lncRNAs displayed positional overlap with previously identified LPS-regulated lncRNA exons from mouse bone marrow-derived dendritic cells [6] and displayed no significant homology. This result is consistent with rapid transcriptional turnover of lncRNAs across species [23] . Our initial differential expression analysis thus revealed a widespread programme of LPS-induced expression changes in a class of RNA molecule that has not been previously studied in primary human monocytes. LncRNAs are associated with an enhancer-like chromatin state Previous studies have reported the presence of transcription at active enhancers marked by H3K4me1 (ref. 18 ). While the poised/active promoter-associated mark, H3K4me3, may also be present at distal enhancer loci [24] , the ratio of H3K4me1/H3K4me3 is commonly used as a discriminatory mark between enhancers and promoters (reviewed in refs 14 , 17 ). To explore whether our differentially expressed lncRNAs represent transcription from enhancer-like regions, we utilized recently available histone modification ChIP-seq data from the ENCODE consortium. We downloaded alignments for H3K4me1 and H3K4me3 ChIP-seq data in CD14+ resting monocytes and assessed the read coverage over intervals surrounding the transcription start site (TSS, ±0.5 Kb) of differentially expressed lncRNAs. An equivalent analysis using differentially expressed protein-coding genes ( n =530) provided a comparison set. To eliminate confounding influences of marks associated with protein-coding genes on lncRNA marks, we removed lncRNAs that either overlapped (that is, antisense) or shared a TSS interval (<2 Kb) with protein-coding genes. 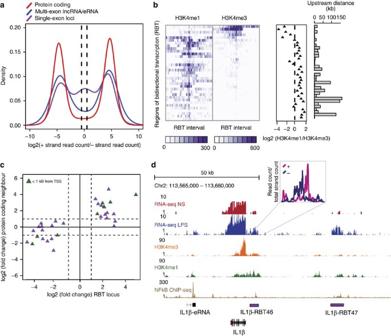Figure 4: Bi-directional transcription defines a second set of eRNAs. (a) Distribution of the ratio of forward strand/reverse strand read counts for monoexonic loci, lncRNAs (including eRNAs) and protein-coding genes. Dashed lines indicate a forward strand/reverse strand ratio of 2. The distribution for monoexonic loci suggests a subset of loci that are transcribed from both DNA strands (ratio<2). (b) H3K4me1 and H3K4me3 profile across differentially expressed RBT. RBT distally located from protein-coding genes display enhancer chromatin signatures. (c) Scatterplot displaying the relationship between the fold changes observed (log2) for RBT and fold changes (log2) for their nearest downstream protein-coding gene. Solid line indicates no change and dashed lines indicate fold changes>2. (d) In addition to a uni-directional eRNA downstream ofIL1β, 2 upstream RBT are regulated by LPS and have evidence for NF-κB binding (lower panel). This resulted in the subsequent analysis of 132/221 lncRNAs (see Supplementary Table 4 online). We hypothesized that a subset of our lncRNAs would display canonical mRNA-like promoter histone signatures (H3K4me1/H3K4me3 low) and a subset, representing enhancer RNAs (eRNAs), would display enhancer-like signatures (H3K4me1/H3K4me3 high). As expected, the majority of differentially expressed protein-coding genes displayed punctate binding of H3k4me3 around the TSS ( Fig. 2a ). In contrast, there was a relatively weaker signal for this histone modification at lncRNA TSS intervals, with only a small subset displaying a high H3K4me3 density ( Fig. 2b ). There was a stronger H3K4me1 signal across intervals for lncRNAs than protein-coding genes, with more dispersed binding around the TSS than for H3K4me3 ( Fig. 2a,b ). To investigate transcripts derived from enhancer regions, we calculated the ratio of H3K4me1/H3K4me3. The distribution of H3K4me1/H3K4me3 for protein-coding genes was markedly different from that of lncRNAs ( Fig. 2a,b ). Protein-coding genes predominantly displayed characteristic promoter marks whereas a large proportion of the investigated lncRNAs were associated with a dominant H3K4me1 histone mark ( Fig. 2a,b ), suggestive of transcription occurring from enhancer regions. Using an H3K4me1/H3K4me3 ratio of >1.2 and <0.8 to define enhancer and promoter states, respectively, we were able to show that 76 lncRNAs (58%) were putative eRNAs, 40 (30%) had canonical promoter signatures and 16 (12%) could not be assigned to either group, that is, 0.8<H3K4me1/H3K4me3<1.2) (see Supplementary Table 4 online). Hereafter, we refer to those RNA transcripts that have higher levels of H3K4me1 compared with H3K4me3 as eRNAs, which differ from canonical lncRNAs (can-lncRNAs), where the reverse is true ( Fig. 2c ). Figure 2: LncRNAs can be distinguished by canonical promoter and enhancer chromatin signatures. ( a ) H3k4me3 and H3K4me1 binding across a 1 Kb interval centred on the transcription start site of expressed protein-coding genes. Profiles are sorted based on the height of the H3K4me3 peak. Also provided is a plot of the H3K4me1/H3K4me3 log2(ratio) at each TSS (mean over interval). ( b ) H3k4me3 and H3K4me1 binding across a 1 Kb interval centred on the transcription start site of differentially expressed lncRNAs. Profiles are sorted on the height of the H3K4me3 peak. Also provided is a plot of the H3K4me1/H3K4me3 log2(ratio) at each TSS (mean). ( c ) Example of a lncRNA with a canonical promoter-like chromatin signature (can-lncRNA, left) and a lncRNA with an enhancer signature (eRNA, right). Figures were produced using the UCSC genome browser. Full size image Correlation between eRNA and local mRNA expression Transcription from enhancers has been linked with the activity of nearby protein-coding loci. To investigate whether monocytic eRNAs were regulated alongside protein-coding genes, we assessed the correlation of fold changes between eRNAs and can-lncRNAs with their closest expressed protein-coding gene neighbours. Although our eRNAs were no closer in proximity to protein-coding genes than can-lncRNAs ( Fig. 3a ), the correlation in fold change (LPS-stimulated versus unstimulated) between eRNAs and their closest protein-coding gene neighbour was stronger than that of can-lncRNAs ( Fig. 3b , r =0.52 and 0.24, respectively). Of particular interest were eRNAs paired with protein-coding genes known to have roles in the monocytic inflammatory response. Such genes included PTGS2, IRF2 ( Fig. 3b ) , ACSL1, MARCKS, IL6 ( Fig. 3b ) , IL10RA, IL10RB and interleukin 1β ( IL1β ) ( Fig. 3b ) (see Supplementary Table 4 online). Figure 3: eRNA expression correlates with protein-coding gene expression. ( a ) Distribution of distances from the closest expressed protein-coding gene for eRNAs and can-lncRNAs. ( b ) Correlation between absolute fold changes for eRNAs and can-lncRNAs with their nearest expressed protein-coding gene neighbour. Full size image Bi-directional transcription at promoter and enhancer regions Bi-directional expression of short transcripts has been described to occur at promoters and distal enhancers in both human and mouse cells [15] , [18] , [25] , [26] . We aimed to exploit the stranded nature of our RNA-seq data in order to define non-coding regions of the genome that were characterized by transcription from both forward and reverse strands. To this end, we merged cufflinks predicted single exon transcripts, regardless of strand, to produce a set of multi-transcript loci. A set of high quality intervals were obtained by only including those that were expressed at an FPKM>1 and had>20 read counts in at least two samples. This resulted in a set of 349 intervals. To address the presence of regions of bi-directional transcription (RBT), we plotted the distribution of the forward strand/reverse strand read count ratio across these intervals. The distribution was tri-modal ( Fig. 4a ), demonstrating that a proportion of intervals represent genomic regions that are transcribed bi-directionally (log2(ratio)~0). This was in contrast to protein-coding genes and can-lncRNAs/eRNAs, whose distributions suggested the predominance of transcription coming from one of either the forward or reverse strand ( Fig. 4a ). In order to identify LPS-regulated RBT, we assessed differential expression across 69 loci that had a forward strand/reverse strand ratio<2 that is, bi-directionally transcribed. Interestingly, none of these regions overlapped lncRNAs from either the Gencode V13 or HumanBodyMap lncRNA catalogues, suggesting that these are a novel set of transcriptional units. 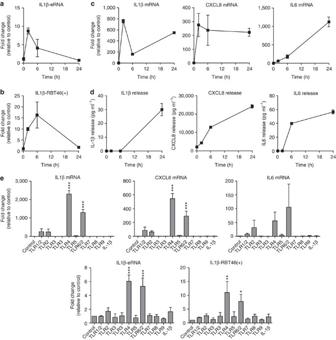Figure 5: Characterisation of LPS-induced lncRNA and mRNA expression. Following exposure of human monocytic THP-1 cells to buffer or 1 μg ml−1LPS, we measured the time course of expression of (a) IL1β-eRNA, (b) IL1β-RBT46(+), (c) IL1β mRNA, CXCL8 mRNA and IL6 mRNA and (d) release of IL1β, CXCL8 and IL6 protein. Subsequent studies determine the expression of IL1β-eRNA, IL1β-RBT46(+), IL1β mRNA, CXCL8 mRNA and IL6 mRNA following 2 h exposure to a range of inflammatory agonists (e). Data are the mean±s.e.m. of three independent experiments. Statistical significance was determined using a one-way analysis of variance with a Dunnett’s post test versus untreated control, where *P<0.05, **P<0.01 and ***P<0.001. Importantly, 35 (51%) RBT were differentially expressed on LPS stimulation (FDR<0.05) (see Supplementary Table 5 online). To characterize these loci further, we examined histone mark profiles across each RBT interval ( Fig. 4b ). A proportion of these loci were marked by high H3K4me3 compared with H3K4me1, which is likely due to their close proximity to protein-coding gene promoters. Indeed, when we removed mRNA-flanking RBTs that are located within 2 Kb of a protein-coding gene TSS ( n =9), we found that 26/26 could be classified as transcribed enhancers (that is, H3K4me1/H3K4me3>1.2). The reason for bi-directional transcription at these loci remains obscure. Nevertheless, we observed a positive correlation between LPS-induced changes in RBT expression and changes in expression of their neighbouring protein-coding gene ( Fig. 4c ). As with our described unidirectional eRNAs, we observed co-regulation of RBT and important regulators of the immune response. For example, TRAF1, IL37, CXCR4, IFNGR2 and CCRN4L ( Supplementary Table 5 ) all have upstream co-regulated RBT. Of particular interest, we identified an mRNA-flanking RBT ( IL1β−RBT46 ) and another within an enhancer region ( IL1β−RBT47 ) located upstream of the important inflammatory mediator, IL1β . Together with our analysis of multi-exonic eRNAs, these data suggest that transcriptional regulation at this locus, and potentially many more, may involve complex regulatory networks that include transcription from both uni- and bi-directionally transcribed enhancers. Figure 4: Bi-directional transcription defines a second set of eRNAs. ( a ) Distribution of the ratio of forward strand/reverse strand read counts for monoexonic loci, lncRNAs (including eRNAs) and protein-coding genes. Dashed lines indicate a forward strand/reverse strand ratio of 2. The distribution for monoexonic loci suggests a subset of loci that are transcribed from both DNA strands (ratio<2). ( b ) H3K4me1 and H3K4me3 profile across differentially expressed RBT. RBT distally located from protein-coding genes display enhancer chromatin signatures. ( c ) Scatterplot displaying the relationship between the fold changes observed (log2) for RBT and fold changes (log2) for their nearest downstream protein-coding gene. Solid line indicates no change and dashed lines indicate fold changes>2. ( d ) In addition to a uni-directional eRNA downstream of IL1β , 2 upstream RBT are regulated by LPS and have evidence for NF-κB binding (lower panel). Full size image LPS-induced lncRNAs are enriched for NFκB binding sites Given the importance of the inflammatory transcription factor (TF) NF-κB in regulating the transcriptional response to infection, we were interested in identifying whether our differentially expressed lncRNAs showed evidence for NF-κB binding. We used the genomic association tester [27] to assess the overlap of eRNA and can-lncRNA promoters (±0.5 Kb around TSS) as well as RBT intervals with TNFα-induced NF-κB binding in lymphoblastoid cell lines. First, we established the overlap between differentially expressed protein-coding promoters and NF-κB. Protein-coding promoters were significantly enriched for NF-κB binding ( Table 1 ), validating the use of this cell type/stimulation procedure for the analysis of lncRNAs. Consistent with immune regulation of can-lncRNAs, we found a significant enrichment for NF-κB binding ( Table 1 ). However, there was no significant overlap between eRNA promoters and NF-κB binding sites ( Table 1 ). To assess whether the difference in NF-κB binding between can-lncRNAs and eRNAs was due to differences in binding location, we also assessed NF-κB binding across gene bodies (TSS-TTS). We found that both eRNAs and can-lncRNAs were enriched for NF-κB binding across their gene bodies ( Table 1 ). We did not see a significant overlap between RBT intervals and NF-κB binding sites, although this may be due to low numbers in this group. Significantly, where we have shown uni- and bidirectional non-coding transcription at the IL1β locus, we also observed coincident NF-κB binding ( Fig. 4d ). This evidence suggests that eRNAs are either regulated by NF-κB themselves, or that they are transcribed from regions that contain NF-κB binding sites important for regulating the expression of nearby mRNA. Table 1 Association of protein-coding genes, can-lncRNAs and eRNAs with NFκB binding. Full size table Characterization of IL1β-eRNA and IL1β-RBT46 expression Having shown widespread changes in the expression of eRNAs, can-lncRNAs and RBTs following LPS stimulation, we wanted to examine whether these regulated the inflammatory response. To this end, we focused upon the production and release of IL1β as a marker of monocyte activation, since this is the second most highly expressed mediator in response to LPS ( Supplementary Table 1 ) and is an important driver of the inflammation associated with the innate immune response [28] . This cytokine is also situated in a region that we have shown to display high transcriptional complexity—it has a downstream eRNA ( IL1β-eRNA ) and an upstream mRNA-flanking RBT ( IL1β-RBT46 ) ( Fig. 4d ). Given the difficulty in transfecting primary human monocytes, these studies were performed in the monocytic THP-1 cell line. For clarity, we have only included the data for the +ve strand of RBT46, since the results with –ve strand were identical. Measurement of the time course showed rapid LPS induction in IL1β-eRNA ( Fig. 5a ) and IL1β-RBT46 (+) ( Fig. 5b ) expression that peaked at ~2 h and ~6 h, respectively. This correlated with that of IL1β mRNA production as well as the generation of two additional, highly expressed inflammatory mediators, CXCL8 and IL6 ( Fig. 5c ). As might be expected, mRNA production preceded the extracellular release of IL1β, CXCL8 and IL6 protein ( Fig. 5d ). Since our studies have focused upon LPS stimulation via TLR4, we also examined the profile of IL1β-eRNA and IL1β-RBT46 (+) expression in response to a range of alternative inflammatory mediators including IL1β and other TLR agonists. These studies showed that IL1β, CXCL8 and IL6 mRNA expression at 2 h was only induced in response to LPS (via TLR4) and FSL-1 (via TLR-2/6), with a small but non-significant increase following exposure to Pam3CSK4 (via TLR-1/2) and HKLM (via TLR-2) ( Fig. 5e ). In the case of IL6 mRNA expression, this early time point meant that the changes were not significant. This selective response is likely to reflect the profile of receptor expression on the monocytic THP-1 cell line. As might be expected if their activation was mediated via similar intracellular pathways, we found that the induction of IL1β-eRNA and IL1β-RBT46 (+) mirrored that of IL1β ( Fig. 5e ) Figure 5: Characterisation of LPS-induced lncRNA and mRNA expression. Following exposure of human monocytic THP-1 cells to buffer or 1 μg ml −1 LPS, we measured the time course of expression of ( a ) IL1β-eRNA, ( b ) IL1β-RBT46(+), ( c ) IL1β mRNA, CXCL8 mRNA and IL6 mRNA and ( d ) release of IL1β, CXCL8 and IL6 protein. Subsequent studies determine the expression of IL1β-eRNA, IL1β-RBT46(+), IL1β mRNA, CXCL8 mRNA and IL6 mRNA following 2 h exposure to a range of inflammatory agonists ( e ). Data are the mean±s.e.m. of three independent experiments. Statistical significance was determined using a one-way analysis of variance with a Dunnett’s post test versus untreated control, where * P <0.05, ** P <0.01 and *** P <0.001. Full size image Having predicted the presence of NF-κB binding sites at the genomic locations of IL1β-eRNA and IL1β-RBT46 , we proceeded to measure NF-κB binding by ChIP in combination with qRT–PCR, using an antibody to the p65 RelA DNA binding subunit. These studies showed a 3.2- and 4.3-fold enrichment in NF-κB binding (relative to non-treated controls) within the promoter regions of IL1β-eRNA and IL1β-RBT46(+) following exposure to LPS, respectively ( Fig. 6a ). This was comparable with the 3.7-fold enrichment seen within the promoter region of the NF-κB regulated chemokine, CXCL8. As predicted by the existing ChIP-seq data in ENCODE, the promoter region of IL1β did not demonstrate NF-κB binding as measured by ChIP–qPCR ( Fig. 6a ). To confirm the ChIP–qPCR data, we examined the action of TPCA-1, an inhibitor of IκB kinase 2 that is an upstream activator of NF-κB [29] . TPCA-1 attenuated the LPS-induced production of IL1β-eRNA , IL1β-RBT46(+) and CXCL8 with an IC 50 of 1.0 μM, 0.9 μM and 1.3 μM, respectively ( Fig. 6b ). TPCA-1-mediated inhibition of NF-κB binding was confirmed using ChIP–qPCR ( Fig. 6a ). Interestingly, despite the absence of NF-κB binding, TPCA-1 attenuated IL1β production, giving an IC 50 of, 0.7 μM ( Fig. 6b ) and suggests that IL1β production might be indirectly regulated through expression of IL1β-eRNA and IL1β-RBT46(+) . 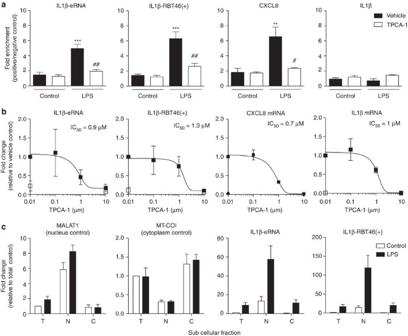Figure 6: NF-κB dependency and subcellular distribution of IL1β-eRNA and IL1β-RBT46(+). NF-κB dependency in human monocytic THP-1 cells was evaluated using TPCA-1, an inhibitor of IKK2. (a) Cells were incubated with TCPA-1 (10 μM) for 30 min prior to stimulation with LPS (1 μg ml−1) for 60 min. ChIP in combination with qRT–PCR was used to detect NF-κB binding within the promoter regions of IL1β-eRNA, IL1β-RBT46(+), CXCL8 and IL1β. Data were expressed as the fold enrichment of negative control primers, amplifying regions of the genome not transcribed or bound by NF-κB in human monocytes. (b) Cells were incubated with TCPA-1 (indicated concentration) for 30 min prior to stimulation with LPS (1 μg ml−1) for 2 h and the expression of IL1β-eRNA, IL1β-RBT46(+), IL1β and CXCL8 mRNA was measured by qRT–PCR. (c) The subcellular distribution was determined by fractionation into total (T), nuclear (N) or cytoplasmic (C) fractions following exposure to buffer or 1 μg ml−1LPS for 2 h. Data are the mean±s.e.m. of three independent experiments. Statistical significance was determined using a one-way analysis of variance with Tukey’s multiple comparisons test, where **P<0.01 and ***P<0.001 versus unstimulated vehicle and#P<0.05 and##P<0.01 versus LPS-stimulated vehicle. Figure 6: NF-κB dependency and subcellular distribution of IL1β-eRNA and IL1β-RBT46(+). NF-κB dependency in human monocytic THP-1 cells was evaluated using TPCA-1, an inhibitor of IKK2. ( a ) Cells were incubated with TCPA-1 (10 μM) for 30 min prior to stimulation with LPS (1 μg ml −1 ) for 60 min. ChIP in combination with qRT–PCR was used to detect NF-κB binding within the promoter regions of IL1β-eRNA, IL1β-RBT46(+), CXCL8 and IL1β. Data were expressed as the fold enrichment of negative control primers, amplifying regions of the genome not transcribed or bound by NF-κB in human monocytes. ( b ) Cells were incubated with TCPA-1 (indicated concentration) for 30 min prior to stimulation with LPS (1 μg ml −1 ) for 2 h and the expression of IL1β-eRNA, IL1β-RBT46(+), IL1β and CXCL8 mRNA was measured by qRT–PCR. ( c ) The subcellular distribution was determined by fractionation into total (T), nuclear (N) or cytoplasmic (C) fractions following exposure to buffer or 1 μg ml −1 LPS for 2 h. Data are the mean±s.e.m. of three independent experiments. Statistical significance was determined using a one-way analysis of variance with Tukey’s multiple comparisons test, where ** P <0.01 and *** P <0.001 versus unstimulated vehicle and # P <0.05 and ## P <0.01 versus LPS-stimulated vehicle. Full size image Much of the previous functional analysis of lncRNAs and eRNAs has suggested that these operate within the nucleus to regulate the transcription of protein-coding mRNAs [12] , [30] . We therefore determined the subcellular localization of IL1β-eRNA and IL1β-RBT46 (+). We assessed the effectiveness of our separation procedure by using MALAT1 lncRNA as a nuclear marker and the mitochondrial cytochrome c oxidase 1 (MT-CO1) as a cytoplasmic marker. Figure 6c demonstrates successful subcellular fractionation, with MALAT1 predominantly associated with the nucleus and MT-CO1 located in the cytoplasmic fraction. There was no significant change in the expression of these markers following exposure to LPS. Interestingly, both IL1β-eRNA and IL1β-RBT46 (+) were predominantly localized in the nucleus of both unstimulated and LPS-stimulated cells ( Fig. 6c ). These data show that LPS-induced IL1β-eRNA and IL1β-RBT46 (+) expression follows a similar time course to that of IL1β , is dependent on the activation of the inflammatory transcription factor NF-κB and if functional, are acting in the nucleus to regulate gene transcription. IL1β eRNA and IL1β RBT46 regulate IL1β expression Given their genomic position ( Fig. 4d ) and nuclear localization ( Fig. 6c ), we speculated that IL1β-eRNA and IL1β-RBT46 might regulate the transcription of IL1β . To examine this hypothesis, we designed a panel of five locked nucleic acid (LNA)-based antisense inhibitors against IL1β-eRNA and IL1β-RBT46 (+) and transfected them into the monocytic THP-1 cells. Following LPS stimulation, we found that in the case of both IL1β-eRNA and IL1β-RBT46 (+), only one (of the five) attenuated lncRNA production ( Fig. 7a ). However, these LNA antisense inhibitors, but not two negative controls, reduced LPS-induced IL1β-eRNA and IL1β-RBT46 (+) generation by 85±9% and 53±9%, respectively ( Fig. 7a ). Of relevance, we also failed to attenuate LPS-induced IL1β-eRNA production using a panel of four siRNAs ( Supplementary Fig. 4a ) despite showing a 64±4% reduction in LPS-induced IL6 mRNA production using a positive control siRNA ( Supplementary Fig. S4b ). In contrast, we were able to show knockdown using all five LNA antisense inhibitors targeted against the constitutively expressed lncRNA, OIP5-mf-lncRNA ( Supplementary Fig. S4c ). These studies suggested that unlike previous reports that have successfully employed both LNA antisense and siRNA for the knockout of constitutively expressed lncRNAs and eRNAs [31] , [32] , [33] , this approach is more problematic when applied to lncRNAs that are located within the nucleus and rapidly induced upon exposure to LPS. 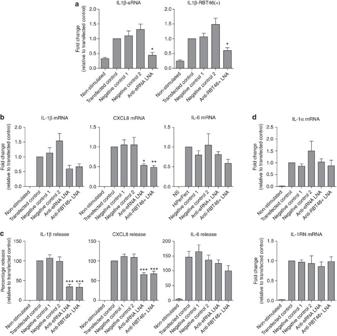Figure 7: IL1β-eRNA and IL1β-RBT46(+) regulate LPS-induced IL1β and CXCL8 expression and release. Human monocytic THP-1 cells (Anti-RBT46+) were transfected with two negative control LNAs or an LNA antisense against either IL1β-eRNA (Anti-eRNA) or IL1(β)-RBT46(+) (Anti-RBT46+) at a final concentration of 30 nM. Cells were then treated with either buffer (non-stimulated) or LPS prior to quantification of (a) IL1β-eRNA1 and IL1β-RBT46(+) expression at 2 h (b) IL1β mRNA, CXCL8 mRNA and IL6 mRNA at 24 h, (c) IL1β, CXCL8 and IL6 protein release at 24 h and (d) IL1α mRNA and IL1RN mRNA at 24 h. Data are the mean±s.e.m. of nine independent experiments. Statistical significance was determined using a one-way analysis of variance with a Dunnett’s post test, where *P<0.05, **P<0.01 and ***P<0.001. Figure 7: IL1β-eRNA and IL1β-RBT46(+) regulate LPS-induced IL1β and CXCL8 expression and release. Human monocytic THP-1 cells (Anti-RBT46+) were transfected with two negative control LNAs or an LNA antisense against either IL1β-eRNA (Anti-eRNA) or IL1(β)-RBT46(+) (Anti-RBT46+) at a final concentration of 30 nM. Cells were then treated with either buffer (non-stimulated) or LPS prior to quantification of ( a ) IL1β-eRNA1 and IL1β-RBT46(+) expression at 2 h ( b ) IL1β mRNA, CXCL8 mRNA and IL6 mRNA at 24 h, ( c ) IL1β, CXCL8 and IL6 protein release at 24 h and ( d ) IL1α mRNA and IL1RN mRNA at 24 h. Data are the mean±s.e.m. of nine independent experiments. Statistical significance was determined using a one-way analysis of variance with a Dunnett’s post test, where * P <0.05, ** P <0.01 and *** P <0.001. Full size image Despite these limitations, we demonstrated that knockdown of IL1β-eRNA and IL1β-RBT46 (+) attenuated LPS-induced IL1β mRNA expression and protein release at 24 h ( Fig. 7b/c ). Thus, we observed a 40 and 35% reduction in IL1β mRNA ( Fig. 7b ) and a 66 and 67% reduction in IL1β protein release ( Fig. 7c ) following inhibition of IL1β-eRNA and IL1β-RBT46( +), respectively ( Fig. 7c ). The effect of IL1β-eRNA and IL1β-RBT46( +) knockdown did not appear to be non-specific since this had no effect upon LPS-induced expression of IL1α and IL1RN ( Fig. 7d ), that are located in the same genomic region or upon expression of the distally located IL6 ( Fig. 7c ). Significantly, we showed a 47 and 52% reduction in CXCL8 mRNA ( Fig. 7b ) that translated into a small but significant reduction of 35 and 33% in CXCL8 protein release ( Fig. 7c ) following inhibition of IL1β-eRNA and IL1β-RBT46( +), respectively ( Fig. 7c ). Overall, this indicates that these LPS-induced IL1β-eRNA and IL1β-RBT46 (+) regulate mRNA expression and downstream release of IL1β and CXCL8 following activation of the innate immune response. To further our knowledge on the potential role of lncRNAs during the activation of the innate immune response, we have used RNA sequencing of ribosomal RNA (rRNA)-depleted, stranded RNA libraries to study the human monocytic response to LPS stimulation. We identified 2,607 lncRNAs using an ab initio transcript assembly. Interestingly, our data support the notion that lncRNA expression is tissue-restricted [34] as we observe 1,318 lncRNAs that have not been previously identified in Gencode [8] or the HumanBodyMap [7] . In addition to these multi-exonic lncRNAs, we uncovered a set of novel bi-directionally transcribed genomic loci (RBT, n =69), a feature of our data that was made possible through stranded RNA sequencing. Previous studies have shown that exposure to LPS induces changes in multiple miRNAs that regulate the innate immune response through targeting the translation of key signalling proteins [10] , [35] . Significantly, we found 221 lncRNAs and 35 RBTs to be differentially expressed in response to LPS and thus may be important in monocyte activation. Examination of the position and homology between these lncRNAs and those previous identified in mouse bone marrow-derived dendritic cells [6] showed virtually no overlap between humans and mice, which is consistent with rapid transcriptional turnover across species [23] . Furthermore, this implies that we must be cautious when extrapolating functional and mechanistic observations between species. As an example, a BLAST search failed to identify the presence in the human genome of the mouse lincRNA-Cox2 that has been reported to regulate the inflammatory response in mouse bone marrow-derived macrophages [20] . Recent investigations in mouse macrophages have indicated that many monocyte lncRNAs are transcribed from enhancer regions [14] , [15] , [36] . In support of this observation, we found that many of the monocyte expressed lncRNAs (58%) are transcribed from regions of the genome that are marked by a high H3K4me1/H3K4me3 ratio, a marker of the existence of enhancer transcription (eRNAs) [37] . In addition, we found that changes in expression of these eRNAs correlated with those of neighbouring protein-coding mRNAs. Mechanistically, this would imply that these eRNAs might act in cis to regulate the expression of their most proximal coding gene, which is consistent with previous data in mouse macrophages [15] . Bi-directional transcription has been shown to be a defining feature of a subset of active enhancers in mouse cortical neurons and human fetal lung fibroblasts [18] , [38] . These non-polyadenylated transcripts are regulated by neuronal activity, a feature that is correlated with activity, regulation of their neighbouring protein-coding gene [18] . We have shown for the first time, the phenomenon of stimulus-dependent bi-directional transcription from both enhancer and promoter regions of activated human monocytes. There is now accumulating evidence that lncRNAs regulate mRNA expression at the level of transcription and translation [12] , [39] . Similarly, recent reports have indicated that eRNAs regulate in cis local mRNA expression in multiple cell types [31] , [40] including mouse macrophages [32] . Having established that LPS induced widespread changes in the expression of lncRNAs and eRNAs in human monocytes that were located close to differentially expressed inflammatory genes, it was important to determine whether these were of functional relevance. Of particular interest for regulation of the innate immune response, was our identification of multiple non-coding transcripts that are situated close to the IL1β gene, an important cytokine that stimulates inflammatory responses in multiple cell types and whose overproduction has been implicated in autoimmune diseases [28] , [41] . These included a downstream eRNA ( eRNA-IL1β-eRNA ) and an upstream mRNA-flanking RBT ( IL1β-RBT46 ). Significantly, we demonstrated that expression of both IL1β-eRNA and IL1β-RBT46 was mediated by the classical proinflammatory transcription factor, NF-κB while knockdown of the IL1β-eRNA and IL1β-RBT46 was shown to attenuate LPS-induced IL1β transcription and protein release. This therefore implies that expression of these lncRNAs regulates the release of this inflammatory mediator and given the genomic position, it might be speculated that they regulate IL1β transcription in cis . However, IL1β-eRNA and IL1β-RBT46 also appear to act in trans since their knockdown inhibited the transcription and release of CXCL8 , albeit to a lesser extent. It is unlikely that this effect was via a non-specific action of the LNA inhibitors since we observed no effect upon LPS-induced expression of IL6 , IL1α and IL1RN . Nevertheless, we cannot rule out the possibility that the effect of CXCL8 is secondary to the inhibition of IL1β, although this is also unlikely as CXCL8 release precedes that of IL1β ( Fig. 5d ). In conclusion, we have shown for the first time that LPS stimulation of primary human monocytes causes widespread changes in lncRNA expression. Crucially, we have demonstrated that the nuclear-located transcripts, IL1β-eRNA and IL1β-RBT46 (+) regulate the transcription and release of the key proinflammatory cytokines, IL1β and CXCL8 although the mechanism is currently unknown. As with miRNAs, we speculate that many of these eRNAs and lncRNAs are important regulators of the innate immune response and future studies will need to focus upon the identification of those that are functionally relevant and the elucidation of their mechanism of action. Treatment of human primary monocytes All human volunteers gave informed written consent as approved by the London–Chelsea NRES ethics committee. Human blood (60 ml) was collected into tubes containing 2% (w/v) EDTA and red blood cells removed by dextran sedimentation. The leukocyte-rich layer was centrifuged at 400 g for 10 min at 4 °C, and the granulocytes were separated from the peripheral blood mononuclear cells (PBMC) fraction using discontinuous Percoll gradients. Percoll fractions of 81, 68 and 55% (v/v) in Dulbecco’s phosphate-buffered saline were prepared and the cell pellet from above was resuspended in 3 ml of 55% (v/v) Percoll and then overlaid onto the pre-prepared gradient. The cells were then separated according to density by centrifugation at 750 g for 25 min at 4 °C. The PBMC were harvested from the 55%/68% interface and then washed with Dulbecco’s phosphate-buffered saline. Monocytes were then isolated from the PBMC fraction using a Miltenyi Monocyte Isolation Kit II according to manufacturer’s instructions. Monocytes were centrifuged and resuspended in RPMI 1640 containing 10% (v/v) fetal calf serum, 10 mg ml −1 (1% (v/v)) penicillin/streptomycin, 2 mM L -glutamine at 1 × 10 6 cells ml −1 and incubated for the times indicated in the absence or presence of 10 ng ml −1 LPS [42] . Experimental samples were treated with 10 ng ml −1 LPS for the indicated time and the controls were left untreated ( n =4 per group). The media was then removed for measurement of CXCL8 and TNFα by ELISA (R&D Systems) and the cells lysed prior to RNA extraction. Culture of human THP-1 cells Monocytic THP-1 cells were obtained from ATCC and cultured in RPMI 1640, supplemented with 10% (v/v) FBS, 1% (w/v) L -glutamine, 1% (w/v) Pen-Strep and 0.1% (v/v) β-mercaptoethanol (Invitrogen Gibco) and incubated in a 37 °C, 5% (v/v) CO 2 humidified incubator. For the time courses, THP-1 cells were stimulated with 1 μg ml −1 LPS ( Escherichia coli 055:B5 , Sigma-Aldrich) for the indicated period of time ( n =3 per group per time point). For all other experiments, THP-1 cells were stimulated with LPS at 1 μg ml −1 for the length of time indicated. Stimulation of THP-1 with TLR agonists THP-1 cells were treated with the following TLR agonists from InvivoGen for 2 h ( n =3 per group) at the concentrations listed; PAM3CSK4 (100 ng ml −1 ), HKLM (10 8 cells ml −1 ), Poly(I:C) (10 mg ml −1 ), Poly(I:C) LMW (10 mg ml −1 ), Flagellin (100 ng ml −1 ), FSL-1 (100 ng ml −1 ), Imiquimod (5 μg ml −1 ), ssRNA40 (1 μg ml −1 ) and ODN2006 (2 μM). THP-1 cells were also treated with buffer as a control, LPS (1 μg ml −1 , E. coli 055:B5 , Sigma-Aldrich) and IL-1β (10 ng ml −1 , recombinant, E. coli , Sigma-Aldrich). RNA isolation Total RNA was extracted using the Qiagen RNeasy kit and included an on-column DNase treatment. RNA used was of high quality (Agilent Bioanalyser (RIN>9.5)). RNA library preparation and sequencing rRNA was depleted using an early-access version of the Ribo-Zero Gold (human/mouse) rRNA Removal Kit (Epicentre). Strand-specific Illumina GA-IIx cDNA libraries were prepared using an early-access version of the ScriptSeq v2 library preparation kit (Epicentre). Two hundred cycles of sequencing on the Illumina GA-IIx instrument were performed to generate 2 × 100 bp paired-end sequencing reads. Quality control of RNA sequencing Quality scores across sequenced reads were assessed using FASTQC v0.9.2 ( http://www.bioinformatics.babraham.ac.uk/projects/fastqc ). All samples were of high quality. The average score (mean and median) at each base across reads in each sample was Q>28. Alignment and transcript assembly Reads were mapped to the human reference genome (Hg19) using TopHat v1.4.0 (ref. 43 ). TopHat first maps to the transcriptome that was supplied as an additional input file. Along with TopHat discovering known splice junctions, a set of known protein-coding junctions (Ensembl 66) were supplied. The following options were used for mapping reads: --mate-inner-dist 60 --num-threads 4 --library-type fr-secondstrand raw-juncs <junctions_file> --transcriptome index <transcriptome index> -n 2 An average of 44.6M reads were mapped (range 40.86–50.82) corresponding to an average of 73.18% (range 69.90–76.05%). Consistent with successful ribosomal RNA (rRNA) depletion, an average of 4.72% (range 1.93–7.32%) of reads mapped to rRNA. Transcripts were assembled for each sample ab initio using Cufflinks v1.3.0 (ref. 1 ) with the following parameterization: --upper-quartile-norm --min-frags-per-transfrag 1 --pre-mrna-fraction 0.5 --junc-alpha 0.001 --overlap-radius 100 Assemblies between samples were compared using Cuffcompare, and transcripts that were present in at least two samples were retained for downstream analysis. Prediction of lncRNAs using RNA sequencing data We utilized the ab initio assembly output from Cufflinks/Cuffcompare in conjunction with the latest human lncRNA annotations (Gencode v13 and the HumanBodyMap [7] to classify transcripts as putative lncRNAs. The outline of the lncRNA prediction pipeline is provided in Fig. 1a . First we removed any transfrags that overlapped ( ⩾ 1 bp on the same strand) transcripts annotated by Ensembl (build 66) as ‘protein_coding’, ‘processed_pseudogene’, ‘unprocessed_pseudogene’, ‘nonsense_mediated_decay’ or ‘retained_intron’. We also filtered any transcripts that overlapped RefSeq annotated coding (CDS) intervals. Next we employed size selection, retaining transfrags that were >200 bp in length and multi-exonic. We then merged our monocyte-derived lncRNA set with the Gencode v13 and the HumanBodyMap [7] sets, producing a non-redundant set of lncRNAs. Assessment of coding potential We used the coding potential calculator (CPC version 0.9-r2) [44] to assess the coding potential of discovered lncRNAs. Abundance estimation and differential expression analysis For correlation analyses, RNA abundance defined as the FPKM was estimated using Cuffdiff V2.0.2. Differential expression analysis was performed using the negative binomial distribution-based method implemented in DESeq [45] on the summed exon read count per gene. Genes were assessed for differential expression if they had an FPKM>1 in either LPS or unstimulated condition (average across replicates). Genes annotated as ‘protein_coding’ in Ensembl (build 66) were used for analysis of protein-coding genes. Multiple testing corrections were performed on a total of 1,065 lncRNAs and 15,020 protein-coding genes using the Q -value method [46] . Profiles of monocyte histone marks across lncRNAs Aligned ChIP-seq data for H3K4me3 and H3K4me1 histone modifications in resting CD14+ monocytes were downloaded from UCSC ENCODE ( http://hgdownload.cse.ucsc.edu/goldenPath/hg19/ENCODEDCC/wgEncodeBroadHistone/ ). Two replicate alignment files for each histone mark were merged using samtools ( http://samtools.sourceforge.net/ ) and profiles were assessed by counting alignments across windows surrounding the transcription start sites of differentially expressed lncRNAs and protein-coding genes (−0.5 to 0.5 Kb) using custom python scripts and BEDTools ( code.google.com/p/bedtools/ ). Heatmaps of the profiles were produced using the heatmap2 (gplots) function in R. Analysis of bi-directional transcription Monoexonic lncRNAs were obtained from our initial cufflinks assembly. Overlapping predictions were merged using BEDTools. This set was filtered, retaining loci that were expressed at an FPKM>1 and were present in at least 2/8 samples with>20 uniquely mapping reads. Bi-directional transcription was assessed by counting the number of reads mapping to the forward and reverse strands. The forward/reverse ratio was used to determine the presence of bi-directional transcription that is, a ratio of 1 would indicate a 50/50 split between sense and antisense transcription. An interval with a ratio of less than twofold was considered bi-directionally transcribed. Differential expression was performed on these loci using DESeq and loci were called differentially expressed at an FDR<0.05. Association of lncRNA loci with NFκB binding sites NF-κB ChIP-seq data (peaks) in TNFα-stimulated lymphoblastoid cell lines were downloaded from UCSC ENCODE ( http://hgdownload.cse.ucsc.edu/goldenPath/hg19/EncodeDCC/wgEncodeHaibTfbs/ ). These data were chosen as the most representative set of TLR4-induced NF-κB binding sites currently available. Binding sites across 10 replicates were merged using BEDTools. Intervals were retained for analysis if they were present (overlapped at least 1 bp with the merged interval) in at least two of the replicate samples. Using lncRNA promoters (defined as a 1 Kb window around the TSS) we assessed the overlap between differentially expressed lncRNAs and NF-κB binding sites. After removing lncRNAs that shared a promoter with protein-coding genes (within 2 Kb of TSS region), we calculated the statistical significance of the overlap using the Genomic Association Tester [27] . Specifically, the base overlap between differentially expressed lncRNA promoters (query set) and NF-κB binding sites was tested against the base overlap between all lncRNA promoters (reference set) from Ensembl annotations, the HumanBodyMap and novel lncRNAs that were expressed in our monocyte samples (average FPKM>1 in either LPS- or unstimulated cells). The expected overlap was computed by randomizing the locations of the query set of intervals among the reference set intervals. From 10,000 randomizations, the procedure computed the expected overlap and an empirical P -value. The reported fold enrichment is the ratio of the observed overlap and the expected overlap. Microarray preparation and data analysis Microarray data were used for validation of differentially expressed protein-coding genes from the RNA-seq analysis. mRNA expression profile was determined using the Agilent SurePrint G3 Human microarrays (v2) following the manufacturer’s instructions. Two channel microarray data were analysed using LIMMA in R-2.14.1. Raw data were processed using Agilent Feature Extraction Software and probes were retained for analysis if they were flagged as being ‘well above background’, ‘not a control probe’ and ‘not saturated’ in at least three arrays. Background correction, within-array robust-spline normalization and between-array quantile normalization were performed using functions in LIMMA. A total of 18,739 probes corresponding to 15,937 genes were analysed for differential expression using the empirical Bayes procedure implemented in LIMMA. Genes were called differentially expressed at an FDR<0.05 and fold change>2. Quantitative PCR validation of lncRNA differential expression Eighteen lncRNAs and eRNAs were chosen for validation ( n =4 per group). Expression of lncRNAs, eRNAs and 18S RNA were determined by qRT–PCR using the SYBR Green PCR mix (Applied Biosystems; primers were obtained from Sigma-Aldrich and are listed in Supplementary Table 6 ). The separate well, 2−(ΔΔCt) method was used to determine relative quantities of individual mRNAs and lncRNAs, which were normalized to 18S RNA. Nuclear and cytoplasmic RNA fractionation THP-1 cells were stimulated with LPS at 1 μg ml −1 for the length of time indicated. The cells were centrifuged and then split into two equal fractions. Total RNA was extracted from one fraction using the normal Qiagen RNeasy protocol while the other fraction was treated with RLN buffer on ice for 5 min, in order to lyse the plasma membrane while leaving the nuclei intact. The nuclei were then isolated by centrifugation at 300 g in a pre-chilled centrifuge. RNA was then extracted from the nuclear and cytoplasm fractions using the normal Qiagen RNeasy protocol. In order to quantify gene expression within the different fractions by qRT–PCR, the 18S values from the total RNA fraction were used to normalize gene expression across all of the fractions. Transfection of THP-1 cells with LNA GAPmers To transfect with LNA GAPmers, THP-1 cells were seeded at 5 × 10 5 cells per well in 24 well plates, in 200 μl of complete growth medium. Transfection mixes were prepared using 190 μl of serum-free growth medium, 10 μl of HiPerFect (Qiagen) plus LNA GAPmers to give a final concentration of 30 nM. Cells were subsequently incubated for 16 h, diluted with 800 μl of complete growth medium and stimulated with LPS. Cells were removed at 2 h and 24 h with the supernatants reserved for analysis of cytokine release. LNA and siRNA sequences are listed in Supplementary Table 7 . Chromatin immunoprecipitation ChIP was performed according to the manufacturer’s guidelines (Active Motif; 53040). In brief, 3 × 10 7 THP-1 cells were stimulated or not with LPS (1 μg ml −1 ) for 60 min. Whole cells were cross-linked with a 1% formaldehyde solution for 15 min at room temperature. Cells were sonicated (Branson Sonifier 250) for two cycles (output: 1, duty cycles: 20%, time: 30 s on 30 s off). DNA concentrations were quantified, and 10 μg of chromatin DNA was used for each ChIP reaction. ChIP assays were performed with 4 μg of antibody (NFκB p65, C-20, Santa Cruz) and incubated overnight at 4 °C, precipitated with agarose beads (supplied) and washed. Bead-bound DNA was reverse cross-linked and purified with DNA Purification columns (supplied). Samples were then analysed by qPCR using the probes listed in Supplementary Table S6 . How to cite this article : Ilott, N. E. et al . Long non-coding RNAs and enhancer RNAs regulate the lipopolysaccharide-induced inflammatory response in human monocytes. Nat. Commun. 5:3979 doi: 10.1038/ncomms4979 (2014). Accession codes : Microarray and RNA-seq data have been deposited in the EBI database ( www.ebi.ac.uk/arrayexpress ) under accession numbers E-MTAB-2408 and E-MTAB-2399 , respectively.